Enriched variations inTEKT4and breast cancer resistance to paclitaxel Among chemotherapeutic agents, paclitaxel has shown great efficacy against breast cancer. Prediction of paclitaxel response may improve patient outcomes. Here we show, using exome sequencing, that in comparison with pre-treatment biopsies, two TEKT4 germline variations are enriched in post-treatment tumours. We find TEKT4 variations in ~\n10% of an independent cohort of 84 pairs of samples. Tektin4 (encoded by TEKT4 ) associates closely with tubulin in doublet microtubules and helps stabilize these structures. These two TEKT4 germline variations in a high cis linkage are biologically relevant, as the ectopic expression of variant TEKT4 deregulates the microtubule stability, antagonizes the paclitaxel-induced stabilizing effect of microtubules and increases paclitaxel resistance. Furthermore, TEKT4 germline variations are associated with reduced disease-free survival and overall survival compared with wild-type TEKT4 in patients undergoing paclitaxel-based chemotherapy. Taken together, we reveal a potential mechanism of resistance to paclitaxel through the acquisition of germline variations in breast cancer. Chemotherapy is the only systemic treatment for certain breast cancer subtypes such as basal-like breast cancers (BLBCs), which are associated with poor clinicopathologic features, a lack of effective treatment targets and poor prognosis [1] . Among chemotherapeutic agents, paclitaxel, which belongs to the group of taxanes (mitotic inhibitors and anti-microtubule agents), has shown great efficacy against breast cancer [2] . Over the past 10 years, the use of anthracycline-based chemotherapy has declined, and the majority of patients with breast cancer are instead receiving taxane-based chemotherapy [3] . The response rate to paclitaxel, however, is 50% as first-line chemotherapy, decreasing to 20–30% when used as second- or third-line chemotherapy [4] ; nearly half of the treated subjects do not respond to paclitaxel. Resistance to paclitaxel has been extensively explored, and various mechanisms have been identified. One potential mechanism is the overexpression of ATP-binding cassette transporters, including P -glycoprotein [5] , [6] and multidrug resistance protein 7 (ref. 7 ). Other possible mechanisms of paclitaxel resistance include the modulation of tubulin [8] , altered expression and structure of microtubule-associated proteins [9] , and activation of anti-apoptotic pathways [10] . However, the predominant mechanism that mediates paclitaxel resistance remains elusive. It is difficult to reliably predict tumour responses to paclitaxel before therapy or to detect when resistance or hypersensitivity develops. Therefore, an improved elucidation of the mechanisms of paclitaxel resistance is required. It is of considerable interest to identify molecular biomarkers in paclitaxel-resistant breast cancer that could provide a more accurate assessment of individual treatment. Paclitaxel-based neoadjuvant chemotherapy (NCT) induces pathologic complete remission in ~\n30% of patients with breast cancer [11] . Although NCT is effective in reducing the size of the primary tumour before surgery, residual disease after NCT is common and is associated with a higher risk of metastatic recurrence compared with patients achieving pathologic complete remission [12] . The altered gene-expression profiles of breast cancer under NCT have been described [13] , [14] , [15] . Recent studies using next-generation sequencing to analyse residual breast cancer after NCT identified diverse pathway activation in drug-resistant tumour cells [16] . However, a comprehensive comparison of the exomes or genomes of pre- and post-NCT samples, especially in breast cancer that underwent paclitaxel-based NCT, has not yet been performed. Here we show that acquisition of genetic variations might occur in breast tumours under paclitaxel-based NCT, and the comparison of the exomes of pre- and post-NCT samples could reveal genetic alterations that are associated with drug resistance, metastatic recurrence and disease progression. This phenomenon, in turn, may lead to the development of targeted therapies, with somatic mutations serving as genomic predictors of tumour response and providing new leads for drug development. TEKT4 variations were enriched after paclitaxel-based NCT Since paclitaxel plays an important role in the chemotherapy of breast cancer, it is of great importance to illustrate the mechanisms of paclitaxel resistance and to identify resistance pathways that can be exploited for therapeutic intervention. 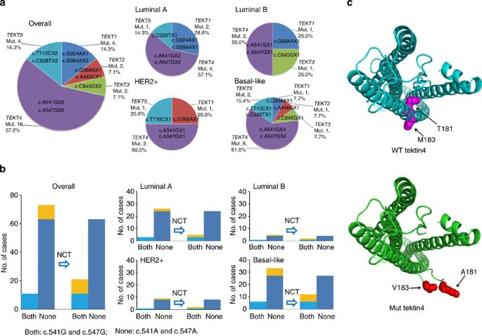Figure 1:TEKTvariations were enriched in breast cancer after paclitaxel-based NCT. (a) The distribution of enrichedTEKTvariations during NCT in 60 breast cancers of four molecular subtypes. The majority of enriched variations (c.A541G and c.A547G) occur inTEKT4. (b) EnrichedTEKT4germline variations (c.A541G and c.A547G) during NCT in 84 breast cancers of four molecular subtypes. The yellow boxes indicate the cases with enrichedTEKT4germline variations after NCT. (c) Wild-type (WT) and mutant (Mut) tektin 4 structures showing the locations of point variations (pink and red spheres). We performed exome sequencing to examine the exomes (~\n100-fold coverage; Supplementary Table 1 ) of two pairs of BLBC samples (pre-treatment biopsies and post-treatment tumours). One pair (P1) is from a 62-year-old Chinese woman, and the other (P2) is from a 58-year-old Chinese woman. Both women were diagnosed with histologically confirmed invasive ductal breast cancer (IDC) and received four cycles of paclitaxel-based NCT (paclitaxel and carboplatin) before undergoing mastectomy [17] , [18] . Each had an ~\n50% reduction in bidimensionally measurable tumour diameter after NCT. Matched biopsy and surgical resection samples were collected before and after NCT. Tumours were confirmed as BLBC [19] , [20] with immunohistochemical phenotypes of ER−, PR−, HER2−, CK5/6+ and EGFR+ by two independent pathologists in the Department of Pathology at the Shanghai Cancer Centre. 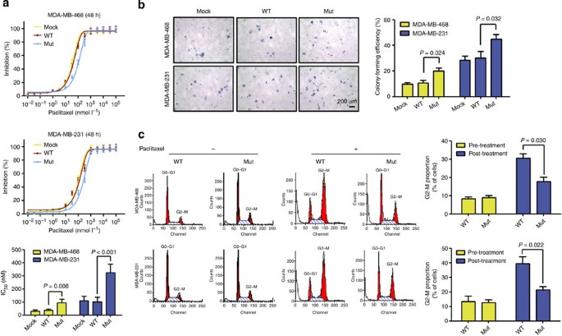Figure 2:TEKT4germline variations induce paclitaxel resistance in breast cancer cells. (a) Cell proliferation was determined by CCK-8 assay after treatment with various concentrations of paclitaxel for 48 h. Mean concentrations of paclitaxel that induce the 50% of cell death (IC50) on mock, wild-type (WT) and mutant (Mut) MDA-MB-468 and MDA-MB-231 cells were calculated and compared (P1=0.008 andP2<0.001 in two-sided Student’sttest). (b) Representative light microscopic images of colonies formed in the soft agar assay with treatment of 50 nM paclitaxel for 48 h. The numbers of colonies were calculated and compared for each group (P1=0.024 andP2=0.032 in two-sided Student’sttest). Scale bar, 200 μm. (c) Flow cytometric analyses of cell cycle distribution in WT and Mut MDA-MB-468 and MDA-MB-231 cells. The proportions of G2-M cells were calculated and compared (P1=0.030 andP2=0.022 in two-sided Student’st-test). Results are the mean±s.d. from three independent experiments. By comparing pre- and post-treatment tumour tissues, we identified 39 somatic single nucleotide variations (SNVs) in P1 and P2 ( Supplementary Table 2 ). These variations were all confirmed by Sanger sequencing. No validated insertions or deletions (indels) were found between pre- and post-NCT tumour tissues in P1 or P2. Upon comparison with pre-treatment biopsies, the analysis of the exome sequence data for P1 and P2 identified and validated the TEKT4 —a gene encoding tektin4, a constitutive protein of microtubules in cilia, flagella, basal bodies and centrioles—as a significantly changed gene (with variations of both c.A541G and c.A547G; Table 1 ) in the post-treatment tumours from both patients. We noticed that there was very low percentage of reads from mutant allele for these two variations in the pre-treatment tumours (~\n3% for P1 and ~\n2% for P2). Whereas, we detected increased percentage of reads from mutant allele in the paired post-treatment tumours (~\n25% for Patient 1 and ~\n30% for Patient 2) and blood DNA (~\n50% for both Patient 1 and 2). Furthermore, we analysed the exome data using LOHcate software ( https://github.com/sidreddy96/lohcate ) to call loss of heterozygosity (LOH). Compared with blood DNA, both of the two pre-treatment tumour samples showed LOH. Tektin4 belongs to the tektin family, which associates closely with tubulin in doublet microtubules and helps stabilize these structures [21] , [22] . We subsequently examined the frequency of enriched TEKT variations in an independent extension cohort of 84 paired samples of different molecular subtypes (clinicopathologic characteristics are listed in Table 2 ). Since there are five members ( TEKT1 - 5 ) in the TEKT family, we performed Sanger sequencing for all five in 60 breast cancer samples ( Fig. 1a ). We identified 28 variations, including four in TEKT1 (14.3%, two cases), two in TEKT2 (7.1%, one case), two in TEKT3 (7.1%, one case), 16 in TEKT4 (57.2%, eight cases) and four in TEKT5 (14.3%, two cases). The majority of the enriched variations among the TEKT family members occurred in TEKT4 . We further sequenced TEKT4 in an additional 24 breast cancer samples and found that after NCT, 74 cases (88.1%) maintained the original genotype ( Supplementary Fig. 1a ), whereas 10 cases (11.9%) enriched both TEKT4 variations c.A541G and c.A547G ( Fig. 1b ). Among the 10 cases, two belong to the luminal A subtype, one belongs to the luminal B subtype, one is HER2+ and six are BLBCs. As controls, we detected these two variations in DNA of blood samples from 200 healthy women and identified the variation rate of 27.0%, which is similar to the results of DNA samples of blood from 84 patients described above ( Supplementary Fig. 1b ), indicating these two variations initially identified in tumour tissues are common (each with minor allele frequency >10%) germline polymorphisms rather than low-frequent somatic changes. Moreover, these two loci were in high cis linkage disequilibrium, as the MAFs of these two SNPs are equal. Table 1 Reads of wild-type and mutant alleles from exome sequencing data. Full size table Table 2 Clinicopathologic characteristics of breast cancer patients who underwent paclitaxel-based neoadjuvant chemotherapy and adjuvant chemotherapy. Full size table Figure 1: TEKT variations were enriched in breast cancer after paclitaxel-based NCT. ( a ) The distribution of enriched TEKT variations during NCT in 60 breast cancers of four molecular subtypes. The majority of enriched variations (c.A541G and c.A547G) occur in TEKT4 . ( b ) Enriched TEKT4 germline variations (c.A541G and c.A547G) during NCT in 84 breast cancers of four molecular subtypes. The yellow boxes indicate the cases with enriched TEKT4 germline variations after NCT. ( c ) Wild-type (WT) and mutant (Mut) tektin 4 structures showing the locations of point variations (pink and red spheres). Full size image Macrodissection alone might not remove all the normal cells. Therefore, we performed microdissection and subsequent pyrosequencing on 56 cases whose pre-, post-treatment tissues and paired blood DNA were available for analysis ( Supplementary Fig. 2 ). 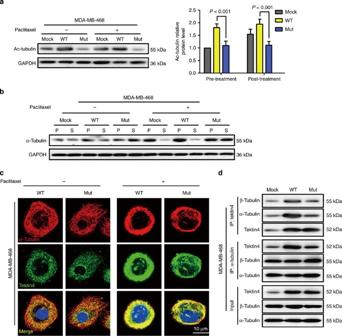Figure 3:TEKT4germline variations reduce microtubule stability and interfere with the interaction between tektin4 and tubulin. (a) The amount of acetylated tubulin was measured by western blotting in mock, wild-type (WT) and mutant (Mut) MDA-MB-468 cells. Relative protein level of Ac-tubulin was calculated and compared (P1,P2<0.001 in two-sided Student’st-test). (b) The tubulin in microtubules (pellet fraction, P) was measured after separating it from free tubulin in the cytosol (supernatant fraction, S) using Western blotting in mock, WT and Mut MDA-MB-468 cells. (c) The colocalization of endogenous α-tubulin (red) and overexpressed tektin4 (green) in WT and Mut MDA-MB-468 cells. Scale bar, 10 μm. (d) Tektin4 or α-tubulin was immunoprecipitated from mock, WT and Mut MDA-MB-468 cells using anti-tektin4 or anti-α-tubulin antibodies, and the immunoprecipitates were immunoblotted with anti-tektin4, anti-α-tubulin or anti-β-tubulin antibodies. Whole-cell lysates were analysed by immunoblotting with anti-tektin4, anti-α-tubulin or anti-β-tubulin antibodies as input. Results are the mean±s.d. from three independent experiments. Full-length images of immunoblots are shown inSupplementary Fig. 8. The results were consistent with our previous findings, that after NCT, 49 cases (87.5%) maintained the original genotype, whereas seven cases (12.5%) enriched both TEKT4 variations c.A541G and c.A547G ( Supplementary Table 3 ). 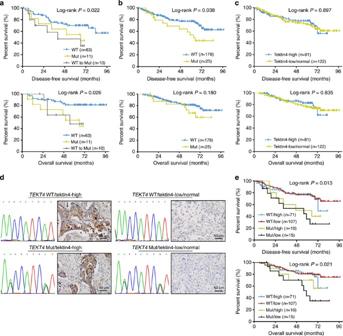Figure 4:TEKT4germline variations are associated with a poor prognosis. (a) Disease-free survival (DFS) and overall survival (OS) in 84 patients who underwent paclitaxel-based NCT, according toTEKT4genotype (P1=0.022 andP2=0.026 in log-rank test). (b) DFS and OS in 203 patients who underwent paclitaxel-based adjuvant chemotherapy, according to the genotype ofTEKT4(P1=0.038 andP2=0.180 in log-rank test). (c) DFS and OS in 203 patients who underwent paclitaxel-based adjuvant chemotherapy, according to the phenotype ofTEKT4(P1=0.897 andP2=0.835 in log-rank test). (d) Representative images ofTEKT4wild-type (WT) and mutant (Mut) genotype based on the Sanger sequencing of patient genomic DNA samples, and representative light microscopic images of tektin4 phenotype by immunohistochemistry using a rabbit polyclonal anti-tektin4 antibody (Proteintech, Chicago, IL, USA; 1:100). Tissue samples of breast cancer were from 203 patients who underwent paclitaxel-based adjuvant chemotherapy. A moderate/strong cytoplasmic staining (stain index (SI)=5–9) was defined as tektin4-high, while a weak or negative staining (SI=0–4) was defined as tektin4-low/normal. Scale bar, 50 μm. (e) DFS and OS in 203 patients who underwent paclitaxel-based adjuvant chemotherapy, according to the combination ofTEKT4genotype and tektin4 phenotype (P1=0.013 andP2=0.021 in log-rank test). Sanger sequencing and pyrosequencing showed excellent consistency in determining the genotype of TEKT4 in pre-, post-treatment tumour tissues and paired blood DNA ( Supplementary Table 4 ). Quantification of mutant alleles via pyrosequencing confirmed the enrichment of TEKT4 variations after NCT ( Supplementary Fig. 3 ). Compared with blood DNA, the pre-NCT tumour samples from the seven cases enriched for TEKT4 variations all showed LOH. However, the germline variations were significantly enriched after paclitaxel-based NCT in the seven cases. Since the tektin4 protein structure visualization predicts that both enriched TEKT4 germline variations (c.A541G, p.T181A and c.A547G, p.M183V) could result in a helix-to-loop structural change ( Fig. 1c ), we speculated that interfering with the interaction between tektin4 and tubulin might produce a varied response to paclitaxel. TEKT4 germline variations induce paclitaxel resistance We further determined that these two TEKT4 germline variations could induce paclitaxel resistance in vitro . First, we examined the levels of tektin4 protein in normal breast MCF-10A cells and various breast cancer cell lines using western blotting ( Supplementary Fig. 4a ). We identified a low expression level of tektin4 in MDA-MB-468 and MDA-MB-231 cells. These two cell lines were determined to be TEKT4 WT by Sanger sequencing. Thus, these two cell lines were selected for the construction of ectopic wild-type (WT; without these two variations) and mutant (Mut; with these two variations) TEKT4 cells. Since the two variations were in high cis linkage disequilibrium due to the proximity of their loci, we overexpressed both of them simultaneously. We then compared the level of tektin4 expression in the virally transduced cells with Hs578T cells, which had high expression level of tektin4 and served as the positive control, to ensure that our experiments were performed under tektin4 levels that were appropriate for breast cancer study ( Supplementary Fig. 4b,c ). Western blotting and real-time reverse transcription PCR (RT-PCR) revealed that the expression of TEKT4 was not affected by the two variations at either protein or mRNA levels. The proliferation of MDA-MB-468 and MDA-MB-231 cells treated with various concentrations of paclitaxel for 48 h was determined by metabolic reduction of WST-8 (CCK-8 cell proliferation assay). The half-maximal inhibitory concentrations (IC 50 ) of paclitaxel on mock, WT and Mut MDA-MB-468 and MDA-MB-231 cells were calculated and compared. The IC 50 values of Mut MDA-MB-468 and MDA-MB-231 cells were 94.7±8.6 nM and 325.0±28.5 nM, respectively, which were approximately threefold higher (results are the mean±s.d. from three independent experiments; P =0.008 for MDA-MB-468 and P <0.001 for MDA-MB-231 in two-sided Student’s t -test) than those of mock or WT cells ( Fig. 2a ). The results of colony formation assays were in accordance with the results of the CCK-8 assays. After treatment with 50 nM paclitaxel for 48 h, Mut cells formed more colonies (approximately twofold, P =0.024 for MDA-MB-468 and ~\n1.5-fold, P =0.032 for MDA-MB-231 in two-sided Student’s t -test) than mock or WT cells, thus showing that these two TEKT4 germline variations increased breast cancer tumour cell resistance to paclitaxel ( Fig. 2b ). Figure 2: TEKT4 germline variations induce paclitaxel resistance in breast cancer cells. ( a ) Cell proliferation was determined by CCK-8 assay after treatment with various concentrations of paclitaxel for 48 h. Mean concentrations of paclitaxel that induce the 50% of cell death (IC 50 ) on mock, wild-type (WT) and mutant (Mut) MDA-MB-468 and MDA-MB-231 cells were calculated and compared ( P 1=0.008 and P 2<0.001 in two-sided Student’s t test). ( b ) Representative light microscopic images of colonies formed in the soft agar assay with treatment of 50 nM paclitaxel for 48 h. The numbers of colonies were calculated and compared for each group ( P 1=0.024 and P 2=0.032 in two-sided Student’s t test). Scale bar, 200 μm. ( c ) Flow cytometric analyses of cell cycle distribution in WT and Mut MDA-MB-468 and MDA-MB-231 cells. The proportions of G2-M cells were calculated and compared ( P 1=0.030 and P 2=0.022 in two-sided Student’s t -test). Results are the mean±s.d. from three independent experiments. Full size image The paclitaxel-resistant phenotype of TEKT4 Mut cells prompted us to determine whether TEKT4 variations are capable of interfering with paclitaxel-mediated mitotic arrest and apoptosis. Flow cytometry revealed that after 48 h of paclitaxel treatment, the majority of WT cells had accumulated at the G2–M phase. In contrast, most of the Mut cells remained in the G1 phase of the cell cycle ( P =0.030 for MDA-MB-468 and P =0.022 for MDA-MB-231 in two-sided Student’s t test; Fig. 2c ). The Mut cells also showed a decreased apoptotic population ( P =0.027 for MDA-MB-468 and P =0.041 for MDA-MB-231 in two-sided Student’s t -test; Supplementary Fig. 5a ). These data consistently indicate that these two TEKT4 germline variations attenuate paclitaxel-induced G2–M arrest and apoptosis in breast cancer cells. To explore the molecular mechanisms underlying the effect of Mut TEKT4 on paclitaxel resistance, we focused on the CDK1–cyclin B1 and Bcl-2 signalling pathways, which have been implicated in the G2–M transition of the cell cycle and in paclitaxel-induced apoptosis [23] . Mock, WT and Mut cells were treated with 50 nM paclitaxel for 48 h, and immunoblotting was performed for markers of mitosis (CDK1, cyclin B1), apoptosis (PARP cleavage) and anti-apoptotic Bcl-2 proteins (Bcl-2, Bcl-xL and Mcl-1). TEKT4 germline variations inhibited the enhanced expression of CDK1 and cyclin B1 after paclitaxel treatment in MDA-MB-468 cells ( Supplementary Fig. 5b ). After paclitaxel treatment, Mut cells exhibited upregulated Bcl-2, Bcl-xL and Mcl-1 levels, resulting in less-cleaved PARP and an increased resistance to apoptosis. In addition, we explored the effect of Mut TEKT4 on cell invasion, cell adhesion, cell cycle distribution and cell proliferation ( Supplementary Fig. 6 ). A Transwell Matrigel invasion assay using conditioned medium as an attractant in the lower chamber revealed no significant effect of Mut on cell invasion ( P =0.893 for MDA-MB-468 and P =0.734 for MDA-MB-231 in one-way ANOVA test; Supplementary Fig. 6a ). As cell–matrix adhesion serves as a key process of tumour cell invasion, we next examined the interaction of WT or Mut cells with the extracellular matrix. However, TEKT4 germline variations had no significant effect on Matrigel adhesion ( P =0.756 for MDA-MB-468 and P =0.784 for MDA-MB-231 in one-way ANOVA test; Supplementary Fig. 6b ). We determined whether TEKT4 variations regulate cell cycle progression in MDA-MB-468 and MDA-MB-231 cells using propidium iodide staining and flow cytometry. The DNA profile of TEKT4 Mut cells was found to be similar to that of control cells ( P =0.683 for MDA-MB-468 and P =0.594 for MDA-MB-231 in one-way ANOVA test; Supplementary Fig. 6c ). Cell proliferation assays also revealed that TEKT4 variations had no significant effect on proliferation ( P =0.724 for MDA-MB-468 and P =0.689 for MDA-MB-231 in one-way ANOVA test; Supplementary Fig. 6d ). Taken together, these data suggest that TEKT4 germline variations lead to paclitaxel resistance in breast cancer cells but have no effect on cell invasion, cell cycle distribution or cell adhesion. TEKT4 germline variations reduce microtubule stability We further investigated the mechanism of paclitaxel resistance induced by TEKT4 germline variations. As a microtubule-associated protein, tektin4 associates closely with the microtubule network and stabilizes these structures. TEKT4 variations might change the protein structure of tektin4, interfere with the interaction of tektin4 and microtubules, and decrease microtubule stability. We therefore explored the effects of WT and Mut TEKT4 on the maintenance of microtubule stability in breast cancer cells. First, we investigated the IC 50 profile of TEKT4 WT and Mut MDA-MB-468 ( Table 3 ) and MDA-MB-231 ( Supplementary Table 5 ) cells for different kinds of agents. Compared with WT MDA-MB-468 cells, Mut cells showed 2.6-fold relative resistance to paclitaxel ( P =0.008 in two-sided Student’s t test), fourfold relative resistance to docetaxel ( P =0.016 in two-sided Student’s t -test) and 2.7-fold relative resistance to epothilone B ( P =0.024 in two-sided Student’s t -test). In contrast, Mut cells were more sensitive to vinblastine, a microtubule-depolymerizing agent (relative resistance=0.2, P =0.041 in two-sided Student’s t -test). No significant difference was observed between WT and Mut cells in resistance to doxorubin, a DNA-damaging agent (relative resistance=0.8, P =0.517 in two-sided Student’s t -test). Furthermore, the drug resistance profile of WT and Mut MDA-MB-231 cells was consistent with that of MDA-MB-468 cells. Table 3 IC 50 profile of wild-type and mutant MDA-MB-468 cells for different kinds of agents. Full size table Since TEKT4 Mut cells were resistant to several microtubule-stabilizing agents (paclitaxel, docetaxel and epothilone B) and were concomitantly sensitive to destabilizing agent (vinblastine), we tested whether the tubulin dynamics in the resistant cells changed. Tubulin that is post-translationally modified by acetylation in microtubules can be extremely stable. According to previous reports, acetylated microtubules can be measured as an indicator of the levels of stable microtubules [24] , [25] . We measured the acetylated microtubules in the cell lysates using an acetylated tubulin-specific antibody ( Fig. 3a ). The results showed that Mut MDA-MB-468 cells have lower levels of acetylated tubulin than mock or WT cells ( P <0.001 for pre-treatment and post-treatment in two-sided Student’s t -test). The tubulin associated with the microtubules (pellet fraction, P) was measured after separating free tubulin in the cytosol (supernatant fraction, S). Mut MDA-MB-468 cells had lower levels of polymerized tubulin compared with mock and WT cells when the cells were grown in the absence of paclitaxel ( Fig. 3b ), suggesting that Mut cells have less-stable microtubules. When the cells were grown in 50 nM paclitaxel, polymerized tubulin increased in each group, especially in the mock and WT cells. We next examined the subcellular localization of recombinant tektin4 and its interaction with tubulin. The immunofluorescence microscopy of MDA-MB-468 ( Fig. 3c ) and MDA-MB-231 cells ( Supplementary Fig. 7 ) overexpressing WT and Mut tektin4 revealed that tektin4 localized to a fibre-like structure in the cytoplasm that completely overlapped with the microtubule labelling produced by an anti-α-tubulin antibody. The pattern of the microtubule network in cells expressing Mut tektin4 changed to a looser structure before and after paclitaxel treatment. Immunoprecipitation assays revealed that the physical connection between tektin4 and α/β-tubulin is weaker in Mut MDA-MB-468 cells ( Fig. 3d ). Together, these results prove that the stabilizing effect of Mut TEKT4 on microtubules is weaker than that of WT TEKT4 . It seems that structural co-crystal and co-interaction studies might demonstrate the altered interactions by Mut TEKT4 in a more direct way. However, these experiments are beyond the scope of current study. Figure 3: TEKT4 germline variations reduce microtubule stability and interfere with the interaction between tektin4 and tubulin. ( a ) The amount of acetylated tubulin was measured by western blotting in mock, wild-type (WT) and mutant (Mut) MDA-MB-468 cells. Relative protein level of Ac-tubulin was calculated and compared ( P 1, P 2<0.001 in two-sided Student’s t -test). ( b ) The tubulin in microtubules (pellet fraction, P) was measured after separating it from free tubulin in the cytosol (supernatant fraction, S) using Western blotting in mock, WT and Mut MDA-MB-468 cells. ( c ) The colocalization of endogenous α-tubulin (red) and overexpressed tektin4 (green) in WT and Mut MDA-MB-468 cells. Scale bar, 10 μm. ( d ) Tektin4 or α-tubulin was immunoprecipitated from mock, WT and Mut MDA-MB-468 cells using anti-tektin4 or anti-α-tubulin antibodies, and the immunoprecipitates were immunoblotted with anti-tektin4, anti-α-tubulin or anti-β-tubulin antibodies. Whole-cell lysates were analysed by immunoblotting with anti-tektin4, anti-α-tubulin or anti-β-tubulin antibodies as input. Results are the mean±s.d. from three independent experiments. Full-length images of immunoblots are shown in Supplementary Fig. 8 . Full size image TEKT4 germline variations associate with patient prognosis It is interesting to see the effect of genotypes and phenotypes of TEKT4 on disease-free survival (DFS) and overall survival (OS) in breast cancer patients who received paclitaxel-containing chemotherapy (clinicopathologic characteristics listed in Table 2 ). Patients with Mut TEKT4 pre-NCT or enriched Mut TEKT4 post-NCT showed significantly worse DFS (log-rank P =0.022) and OS (log-rank P =0.026) than their counterparts with WT TEKT4 ( Fig. 4a ). These associations were also observed in the adjuvant chemotherapy group, in which the Mut genotype of TEKT4 was significantly correlated with worse DFS (log-rank P =0.038) compared with the WT genotypes ( Fig. 4b ), although this effect was not observed between tektin4-high and tektin4-low/normal groups ( Fig. 4c ). We further divided the adjuvant chemotherapy group into four subgroups ( Fig. 4d ): TEKT4 WT/tektin4-high, TEKT4 WT/tektin4-low, TEKT4 Mut/tektin4-high and TEKT4 Mut/tektin4-low. Interestingly, patients with Mut TEKT4 genotype, either with tektin4-low/normal or tektin4-high phenotype, exhibited a worse DFS (log-rank P =0.013) and OS (log-rank P =0.021) than other two groups ( Fig. 4e ). Figure 4: TEKT4 germline variations are associated with a poor prognosis. ( a ) Disease-free survival (DFS) and overall survival (OS) in 84 patients who underwent paclitaxel-based NCT, according to TEKT4 genotype ( P 1=0.022 and P 2=0.026 in log-rank test). ( b ) DFS and OS in 203 patients who underwent paclitaxel-based adjuvant chemotherapy, according to the genotype of TEKT4 ( P 1=0.038 and P 2=0.180 in log-rank test). ( c ) DFS and OS in 203 patients who underwent paclitaxel-based adjuvant chemotherapy, according to the phenotype of TEKT4 ( P 1=0.897 and P 2=0.835 in log-rank test). ( d ) Representative images of TEKT4 wild-type (WT) and mutant (Mut) genotype based on the Sanger sequencing of patient genomic DNA samples, and representative light microscopic images of tektin4 phenotype by immunohistochemistry using a rabbit polyclonal anti-tektin4 antibody (Proteintech, Chicago, IL, USA; 1:100). Tissue samples of breast cancer were from 203 patients who underwent paclitaxel-based adjuvant chemotherapy. A moderate/strong cytoplasmic staining (stain index (SI)=5–9) was defined as tektin4-high, while a weak or negative staining (SI=0–4) was defined as tektin4-low/normal. Scale bar, 50 μm. ( e ) DFS and OS in 203 patients who underwent paclitaxel-based adjuvant chemotherapy, according to the combination of TEKT4 genotype and tektin4 phenotype ( P 1=0.013 and P 2=0.021 in log-rank test). Full size image Furthermore, adjusted hazard ratios (HazRs) with 95% confidence intervals (CIs) were calculated using Cox proportional hazards models ( Table 4 ). For instance, in the NCT group, we observed that clinical response (HazR=7.64, 95% CI: 2.32–18.91, P =0.018 in multivariate Cox regression analysis) and TEKT4 genotype (HazR for WT=5.01, 95% CI: 1.17–10.82; HazR for WT-to-Mut=6.12, 95% CI: 1.26–12.48, P =0.043 in multivariate Cox regression analysis) were independent prognostic factors for DFS after multivariate adjustment. In the adjuvant chemotherapy group, the adjusted use of a multivariate Cox regression revealed that node status (HazR=1.59, 95% CI: 1.02–2.47, P =0.041 in multivariate Cox regression analysis), TEKT4 genotype (HazR=4.05, 95% CI: 1.82–10.2, P =0.021 in multivariate Cox regression analysis) and the combination of TEKT4 genotype and phenotype (HazR=4.77, 95% CI: 1.93–12.71, P =0.012 in multivariate Cox regression analysis) were significant independent prognostic factors for DFS. We also studied the relationship between genotype (WT, Mut and WT-to-Mut) and clinical response to NCT using χ 2 test ( Supplementary Table 6 ). Patients with Mut or WT-to-Mut genotypes have significantly lower partial response (PR) rates than those with the WT genotype. In summary, the patients with Mut genotypes seemed to be resistant to paclitaxel-based chemotherapy and showed a worse survival relative to their WT counterparts. Table 4 Multivariate analysis of disease-free survival in the neoadjuvant chemotherapy and adjuvant chemotherapy cohorts. Full size table The notion that most cancers are ecosystems of subclones has been widely accepted and has implications for clinical applications [26] . While intertumoral [27] , [28] and intratumoral [29] , [30] genetic heterogeneity had been previously demonstrated in cancer, our use of exome sequencing-based algorithms enabled a more comprehensive study of mutation shift after NCT and its clinical impact. In this study, we present evidence that enriched TEKT4 germline variations (c.A541G and c.A547G) during NCT deregulate microtubule stability and result in paclitaxel resistance. Our data suggest that acquisition of genetic variations can occur during chemotherapy, and Mut TEKT4 leads to a poorer response to NCT and poorer survival of patients treated with paclitaxel. For patients carrying these two germline variations in TEKT4 , taxanes may have limited efficacy. Tektins associate closely with tubulin in doublet microtubules via direct, tight and specific interactions [22] . In doublet microtubules, tektins also help to organize the longitudinal spacing of accessory structures, such as groups of inner dynein arms and radial spokes [21] . As a microtubule-associated protein, tektin4 colocalizes with the microtubule network and helps to stabilize these structures [31] . TEKT4 variations might induce an abnormal structure of tektin4 and alter the interaction between tektin4 and microtubules, resulting in reduced microtubule stability. In this report, we proposed that TEKT4 variations (c.A541G and c.A547G) lead to structural changes in tektin4, thus impairing the interaction of tektin4 with microtubules and reducing the stability of microtubules. The decreased stability of the microtubules requires increased concentrations of drug to maintain efficacy and can increase paclitaxel resistance. This finding was further proven by clinical data showing that Mut TEKT4 leads to a poorer response to NCT and reduced survival of patients treated with paclitaxel. An important question addressed here is how NCT treatment affects mutation status in breast cancer, resulting in altered genomics after NCT. We propose that in paclitaxel-treated samples, cytotoxic therapy typically removes the paclitaxel-sensitive subclones ( TEKT4 WT cells) and consequently shifts the landscape in favour of the paclitaxel-resistant subclones ( TEKT4 Mut cells) [32] . Thus, TEKT4 Mut cells probably benefit more from treatment and would exhibit rapid outgrowth [33] . Such information might eventually guide the selection of therapies to prevent the expansion of paclitaxel-resistant subclones [34] . The elucidation of clonal genotypes that are responsive or resistant to treatment provides a basis for determining which combinations of drugs will be effective in preclinical and clinical studies. In our study, we found that c.A541G and c.A547G in TEKT4 were in high cis linkage disequilibrium due to the proximity of their loci. Interestingly, we noticed that in ~\n10% cases of the NCT cohort, TEKT4 variations occurred in post-NCT tumour tissues and paired blood DNA but not in pre-NCT tumour tissues. This finding might be explained by LOH [35] , [36] or an allelic imbalance [37] , [38] during tumorigenesis as well as tumour development. We propose that WT homozygous tumour cells have an advantage in cell growth and formed the majority of the tumour. However, Mut homozygous or heterozygous tumour cells are relatively more resistant to paclitaxel and ultimately predominated within the tumour environment under the selection of paclitaxel. Yet, the mechanisms of the enrichment or selection of these variations are complex and warrant further investigation. One of the limitations of the current study is the relatively small sample size, especially for the NCT cohort. Future studies will be needed to validate the role of TEKT4 germline variations in a larger population. Furthermore, more research is required to elucidate the mechanism by which tektin4 confers microtubule stability and to clarify a possible role in the regulation of the post-translational modification of tubulin. In addition, the effects of TEKT4 germline variations on drug resistance to other agents should be investigated. In conclusion, the comparison of patient exomes and genomes pre- and post-NCT identified functional TEKT4 variations and the destabilization of microtubules in breast cancers given NCT. The identification of TEKT4 germline variations as biomarkers for the prediction of treatment response and prognosis may help us to optimize patients’ options for sequential therapy and thus improve their survival. Further studies based on these findings will help to illustrate drug-resistance mechanisms and identify resistance pathways that can be exploited for therapeutic selection. Human tissues Two cases of typical BLBCs were selected for exome sequencing. P1 is a 62-year-old Chinese woman and P2 is a 58-year-old Chinese woman. These patients were both diagnosed with histologically confirmed IDC and underwent four cycles of paclitaxel-based NCT (paclitaxel and carboplatin) before mastectomy. After NCT, both P1 and P2 had an ~\n50% reduction in bidimensionally measurable tumour diameter. Matched biopsy and surgical resection samples were collected before and after NCT. Tumour tissues were macrodissected to avoid the influence of necrotic or stromal tissues (<5%) resulting from NCT. Tumours were confirmed as BLBC [19] , [20] with an immunohistochemical phenotype of ER−, PR−, HER2−, CK5/6+ and EGFR+ by two independent pathologists in the Department of Pathology of Fudan University Shanghai Cancer Centre (FDUSCC, Shanghai, China). Patients’ menopausal status, lymph node status, grades, chemotherapeutic agents and prognosis were well matched. In addition, two validation cohorts of female patients with IDC were enrolled in this study. Only those patients with operable unilateral tumour and without any evidence of metastasis at diagnosis were enrolled. All patients were treated at FDUSCC between 1 January 2003 and 31 December 2009. Follow-up was completed on 31 March 2013. The median length of follow-up was 61 months (range, 6 to 97 months). Our definition of DFS events included: the first recurrence of disease at a local, regional or distant site; the diagnosis of contralateral breast cancer; and death from any causes [39] . The OS was calculated from the date of diagnosis to the date of death or last follow-up. Patients without events or death were censored at the last follow-up. The clinicopathologic characteristics of patients are listed in Table 2 . In general, both cohorts were well balanced for baseline characteristics. The first cohort consisted of 84 patients with histologically confirmed IDC who had undergone four cycles of paclitaxel-based NCT (paclitaxel and carboplatin). Matched biopsy and surgical resection samples were collected before and after neoadjuvant treatment. The second cohort consisted of 203 patients with histologically confirmed IDC who had received prior surgical resection and paclitaxel-based chemotherapy. Tumour tissues were macrodissected to avoid the influence of stromal tissues (<5%). The molecular subtypes of breast cancer according to immunohistochemical profiles were categorized as follows: luminal A=ER+ or PR+, HER2− and Ki67<14%; luminal B=ER+ or PR+ and HER2+ or Ki67≥14%; HER2+=ER−, PR− and HER2+; and basal-like=ER−, PR−, HER2− and CK5/6+ or EGFR+ (refs 19 , 20 ). Tumours with immunohistochemical phenotypes of ER−, PR−, HER2−, CK5/6− and EGFR− were excluded. The staining and the interpretation of ER, PR, HER2, Ki67, CK5/6 and EGFR have been previously described [19] , [40] . Study approval The use of human tissue samples and clinical data was approved by the Ethical Committee of FDUSCC, and each participant signed an informed consent document. Tumour samples and paired blood samples were obtained from patients undergoing surgical treatment at FDUSCC in accordance with the FDUSCC Institutional Review Boards. Exome capture and sequencing DNA extracted from tumour samples and paired blood samples were sent to Beijing Genomics Institute-Shenzhen for exome sequencing [41] , [42] , [43] . Exome capture was performed using the SureSelect Human All Exon Kit (Agilent, Santa Clara, CA, USA), guided by the manufacturer’s protocols. In brief, the qualified genomic DNA samples were randomly fragmented to 200–500 bp in size, followed by end-repair, A-tailing and paired-end index adapter ligation. Final libraries were validated by Bioanalyser analysis (Agilent, Santa Clara, CA, USA) and quantitative PCR. Each captured library was loaded on the Hiseq 2000 platform, and paired-end sequencing was performed with read lengths of 90 bp, providing at least 100 × average depth for each sample. SOAPaligner 2.20 (ref. 44 ) was used to align the reads to human reference hg19 with parameters set to ‘-a -b -D -o -v 2 -r 1 -t -n 4′. Reads that aligned to the designed target region (TR) were collected for SNV identification and subsequent analysis. For SNV calling, the Variant Quality Score Recalibration method, which builds an adaptive error model using known variant sites, was applied to estimate the probability that each variant is a true genetic variant or a machine artefact. For indel calling, Burrows–Wheeler Aligner (BWA, V.0.5.8) was used to gap align the sequence reads with default parameters to the human reference hg19. GATK IndelRealigner was used to perform local realignment of the BWA-aligned reads and GATK IndelGentotyperV2 was used to call indels. The variants were functionally annotated using an in-house pipeline and were subsequently categorized into missense, nonsense, read-through or splice-site mutations and coding indels, which are likely to be deleterious compared with synonymous and non-coding mutations. Sanger sequencing and protein structure visualization The detection of mutations in frozen tumour tissues and paired blood DNA was performed by Sanger sequencing. PCR amplification was performed on an ABI 9700 Thermal Cycler using standard conditions. After the amplification, products were purified using a QIAquick PCR Purification Kit (Qiagen, Valencia, CA, USA) and directly sequenced on ABI PRISM 3730 automated sequencer (Invitrogen, Carlsbad, CA, USA). Detected mutations were confirmed by re-sequencing of tumour and matched normal blood DNA from new PCR product. The visualization of protein structures was conducted using PyMol (DeLano Scientific, San Carlos, CA, USA). Laser-captured microdissection and LOH detection For each case, one section 15 μm in thickness was stained with hematoxylin and eosin and microdissected using the AS Laser Microdissection system (Leica Microsystems, Wetzlar, Germany). In total, 30–40 tumour foci, each containing ~\n100 cancer cells, were obtained. QIAamp DNA Mini Kits (Qiagen, Valencia, CA, USA) were used to extract DNA from the tissues. The quality and concentration of the extracted DNA were determined using a NanoDrop 2000 (Thermo Fisher Scientific, Wilmington, DE, USA). LOH at the c.A541G and c.A547G sites in the 10 cases enriched with TEKT4 variations was quantitatively assayed by using pyrosequencing technology basically as described previously [45] , [46] . Primer sequences were as follows: forward, GGAAGCCGAGCTCATCCG; biotinylated reverse, CCGGATCTGGCTCACTGCTT; sequencing, GGAGCTGCTGAAGAGA. Allele frequencies were outputted as relative percentages using the Biotage PSQ software, and genotypes were assigned based on the relative allele percentage between blood and paired tumour samples. Informative calls were evaluated as relative ratios of 50:50±10%. LOH was determined as ratios 90:10 or greater in the tumour sample with an informative ratio in the blood sample. Cell cultures Breast cancer cell lines (MDA-MB-468, MDA-MB-231, MCF7, ZR-75-1, BT-474, MDA-MB-435, SK-BR-3 and Hs578T), normal breast MCF-10A cells and 293T cells were obtained from the American Type Culture Collection (Manassas, VA, USA) and maintained in complete growth medium as described previously [39] , [47] . Liquid nitrogen stocks were created upon receipt, and cells were maintained until the start of each study. Cell morphology and doubling times were also regularly recorded to ensure the maintenance of phenotypes. Cells were used for no more than 6 months after being thawed. Western blotting Equal amounts of cell lysates were resolved by SDS–PAGE and transferred to PVDF membranes (Roche, Basel, Switzerland). Blocking was performed for 60 min with 5% non-fat dry milk in TBST, and blotting was performed with primary antibodies for 12–16 h at 4 °C. Primary antibodies included: rabbit polyclonal anti-tektin4 (Abcam, Cambridge, MA, USA; 1:1,000), rabbit polyclonal anti-CDK1 (Santa Cruz Biotechnology, Santa Cruz, CA, USA; 1:1,000), rabbit polyclonal anti-cyclin B1 (Cell Signaling, Beverly, MA, USA; 1:1,000), rabbit monoclonal anti-Bcl-2 (Cell Signaling; 1:1,000), rabbit polyclonal anti-Bcl-xL (Cell Signaling; 1:1,000), rabbit polyclonal anti-Mcl-1 (Cell Signaling; 1:1,000), rabbit polyclonal anti-cleaved PARP (Cell Signaling; 1:1,000), mouse monoclonal anti-α-tubulin (Bioworld, Dublin, OH, USA; 1:1,000), mouse monoclonal anti-β-tubulin (Bioworld, Dublin, OH, USA; 1:1,000), rabbit polyclonal anti-acetylated tubulin (Sigma-Aldrich, Natick, MA, USA; 1:3,000), rabbit polyclonal anti-Flag (Sigma-Aldrich, Natick, MA, USA; 1:3,000) and rabbit polyclonal anti-GAPDH (Cell Signaling; 1:2,000). After extensive washing with TBST, the membranes were incubated for 1.5 h at room temperature with HRP-conjugated goat anti-rabbit antibody (Santa Cruz Biotechnology; 1:3,000), goat anti-mouse antibody (Santa Cruz Biotechnology; 1:2,000), and signal was detected by enhanced chemiluminescence substrate (Pierce Biotechnology). For quantification, the western blot films were scanned and were analysed using ImageJ Version 1.33u software (National Institutes of Health, Bethesda, MD, USA). Plasmids The LV-FLAG lentivirus vector was kindly provided by Dr Jian-Hai Jiang of Fudan University. For the ectopic expression of WT or Mut TEKT4 , the LV-TEKT4-FLAG plasmid was constructed by inserting full-length WT or Mut human TEKT4 cDNA into the LV-FLAG lentivirus vector between BamHI and AgeI sites. TEKT4 variations (c.A541G and c.A547G) were created using Takara MutanBEST mutagenesis kit (TaKaRa, Tokyo, Japan). Mutated constructs were examined by Sanger sequencing, and the correctly modified ones were selected for further experiments. Lentivirus infection and generation of stable cell lines Briefly, using calcium phosphate transfection, 293T cells were co-transfected with lentivirus vectors and the packaging vectors RRE, REV and RSVG. Two days following transfection, viral supernatants were collected, filtered and concentrated by ultracentrifugation. Polybrene (Sigma-Aldrich, Natick, MA, USA) was added at a working concentration of 8 μg ml −1 . Cells were incubated with virus for 12–24 h, washed with phosphate-buffered saline (PBS) and incubated in fresh media. Cell lines were subjected to puromycin selection for 14 d and ectopic expression was verified by real-time RT-PCR and western blot analysis for tektin4. Cells infected with the empty LV-FLAG lentivirus vector were defined as the Mock control. Measurement of cell proliferation Mock, WT and Mut MDA-MB-468 and MDA-MB-231 cells (5 × 10 3 per well) were seeded in 96-well plates. After 6 h, cells were treated with indicated concentration of paclitaxel, respectively. In parallel, 5 × 10 3 cells per well were seeded in 96-well plates and treated with PBS. Cell proliferation was determined by CCK-8 assay as described previously [48] . Soft agar colony formation assay Cells (1 × 10 5 ) were suspended in growth medium containing 0.4% agar. The cells were then plated into a dish containing a hard agar base composed of growth medium and 0.75% agar. The cultures were returned to the incubator and fed every two days with 500 μl of normal growth medium. The photomicrographs of colonies were taken 14 to 21 days later [49] . A colony is defined as a cluster of at least 50 cells. The colony-forming efficiency was calculated as the number of colonies divided by the number of cells plated (%) [50] . Cell invasion and adhesion assay For the Boyden chamber invasion assay, cells were added to the upper compartment of the chamber and 800 μl of medium (containing 0.1% bovine serum albumin) was added into the lower chamber. Cells were incubated and allowed to migrate through Matrigel (BD Biosciences, Bedford, MA, USA) for 24 h. After removal of non-migrated cells, cells that had migrated through the filter were counted. For the cell adhesion assay, the cell suspensions (2.5 × 10 5 in 0.5 ml medium per well) were added to microculture wells precoated with Matrigel (BD Biosciences). The cultures were incubated at 37 °C for 60 min. The wells were washed four times with PBS to remove unattached cells and then the attached cells were stained with 0.5% Crystal Violet in 20% methanol for 30 min. After washing with water, the stained cells were lysed with 30% acetic acid and the absorbance of the lysates was measured at 590 nm. Cell proliferation assay Cell proliferation was quantified by metabolic reduction of WST-8 (CCK-8 cell proliferation assay) to generate a growth curve over 6 days. Mock, WT and Mut MDA-MB-468 and MDA-MB-231 cells were seeded at 2 × 10 4 cells per well in a 96-well plate (day 0) and incubated for a further 3 days. On each successive day, cell proliferation per well was determined by CCK-8 assay. Measurement of tubulin in microtubules Cells were grown in duplicate wells of 24-well dishes to 80% confluence and remained untreated or were treated overnight with 50 nM paclitaxel for 48 h. The tubulin in microtubules was measured as described previously [51] . Briefly, the cells were lysed in a microtubule-stabilizing buffer. The lysates were centrifuged at 10,000 g for 20 min to obtain pellet fractions containing microtubules and supernatant fractions containing soluble tubulin. The proteins in each fraction were precipitated with five volumes of acetone, precipitates were centrifuged and pellets were air-dried. The pellets were resuspended in SDS–PAGE sample buffer, and western blotting analysis of electrophoresed proteins was performed using the indicated antibodies. Measurement of acetylated tubulin To determine the relative amounts of acetylated tubulin, WT and Mut cell lines were grown to 80% confluence in 35-mm dishes and lysed with 1% SDS. Proteins were precipitated by adding five volumes of acetone, and the precipitate was collected by centrifugation for 5 min at 10,000 g . The pellet was dissolved in SDS sample buffer, and western blotting analysis of electrophoresed proteins was performed using indicated antibodies. Immunofluorescence Cells grown on glass coverslips were fixed with 4% paraformaldehyde in PBS for 20 min, permeabilized in 0.3% Triton X-100 in PBS for 10 min, blocked with 5% serum in PBS for 1–2 h and then probed overnight at 4 °C with primary antibodies. Primary antibodies include mouse monoclonal anti-α-tubulin (Bioworld, Dublin, OH, USA; 1:50) and rabbit polyclonal anti-tektin4 (Proteintech, Chicago, IL, USA; 1:50). The coverslips were washed three times with PBS for 10 min, and detection was performed using the appropriate fluorescent secondary antibodies (Invitrogen, Carlsbad, CA, USA) for 60–90 min at room temperature. Nuclei were counterstained with DAPI. Coverslips were mounted on glass slides and viewed using a confocal microscope. Co-immunoprecipitation Briefly, cells (3 × 10 6 ) were collected and lysed in a modified RIPA buffer (1% Triton X-100, 50 mM Tris (pH=7.4), 150 mM NaCl, 2 mM EDTA, protease inhibitor cocktail, 60 mM β-glycerophosphate, 0.2 mM Na 3 VO 4 , 1 mM NaF). Proteins were co-immunoprecipitated with anti-α-tubulin (Cell Signaling) or anti-tektin4 antibody (Proteintech), and western blotting analysis of electrophoresed proteins was performed using indicated antibodies. Whole-cell lysates were analysed by immunoblotting with anti-tektin4, anti-α-tubulin or anti-β-tubulin antibodies as input. Immunohistochemistry Paraffin-embedded sections were deparaffinized and rehydrated. Antigens were retrieved by boiling sections in Tris-EDTA buffer (pH 9.0) at 121 °C for 10 min. After the endogenous peroxidase was blocked by incubating with 3% H 2 O 2 solution in PBS for 10 min, sections were blocked with 5% normal serum and were incubated with rabbit polyclonal anti-tektin4 (Proteintech; 1:100) at room temperature for 2 h. After extensive washing in TBST buffer (25 mM Tris–HCl (pH 7.4), 150 mM NaCl, 0.1% Tween-20), sections were incubated for 60 min with HRP-conjugated goat anti-rabbit secondary antibody (Santa Cruz Biotechnology; 1:200). The immunoreactivity was visualized with 3,3'-diaminobenzidine (Dako, Glostrup, Denmark). Sections were counterstained with haematoxylin (Sigma-Aldrich). The images were captured using the Motic Image Advanced 3.2 image analysis system. Slides were concurrently evaluated by two independent pathologists in the Department of Pathology of FDUSCC. A granular cytoplasmic stain was defined as positive. Briefly, the staining index (SI, range 0–9) was calculated as the result of the intensity score (0, no staining; 1+, faint/equivocal; 2+, moderate; 3+, strong) and the distribution score (0, no staining; 1+, staining of <10% of cells; 2+, between 10 and 50% of cells; and 3+, staining of >50% of cells) [52] . For tektin4 protein in this study, a moderate/strong cytoplasmic staining (SI=5–9) was defined as tektin4-high, while a weak or negative staining (SI=0–4) was defined as tektin4-low/normal [53] , [54] . Statistical analysis All experiments were repeated at least three times. All numerical data were expressed as the mean±s.d. The data were analysed using two-sided Student’s t -test or a one-way ANOVA test. Comparisons of patient and tumour characteristics were performed using the χ 2 test. Survival curves were constructed using the Kaplan–Meier method, and the univariate survival difference was determined with the log-rank test. Adjusted HazRs with 95% CIs were calculated using Cox proportional hazards models. All statistical analysis was performed using Stata statistical software, version 10.0 (StataCorp, College Station, TX, USA). A two-sided P <0.05 was considered statistically significant. Accession codes: The exome sequencing data have been deposited in the GenBank/EMBL/DDBJ BioProject database under the accession code PRJNA243169 . How to cite this article: Jiang, Y.-Z. et al. Enriched variations in TEKT4 and breast cancer resistance to paclitaxel. Nat. Commun. 5:3802 doi: 10.1038/ncomms4802 (2014).